Ionic field effect and memristive phenomena in single-point ferroelectric domain switching Electric field-induced polarization switching underpins most functional applications of ferroelectric materials in information technology, materials science and optoelectronics. Recently, much attention has been focused on the switching of individual domains using scanning probe microscopy. The classical picture of tip-induced switching, including formation of cylindrical domains with size, is largely determined by the field distribution and domain wall motion kinetics. The polarization screening is recognized as a necessary precondition to the stability of ferroelectric phase; however, screening processes are generally considered to be uniformly efficient and not leading to changes in switching behaviour. Here we demonstrate that single-point tip-induced polarization switching can give rise to a surprisingly broad range of domain morphologies, including radial and angular instabilities. These behaviours are traced to the surface screening charge dynamics, which in some cases can even give rise to anomalous switching against the electric field (ionic field effect). Development of modern civilization is inherently enabled by technologies to manipulate and control information. The general theoretical underpinning of information theory was laid as early as middle of nineteenth century and perfected in the middle of twentieth century by Shannon, Neumann and many others [1] . The practical implementation followed a complex path evolving from mechanical platforms to vacuum tubes, and have finally found its present implementation in modern semiconductor devices [2] , [3] . In the last several years, much theoretical and applied interest has been attracted to information technology devices using non-electronic degrees of freedom. Some of the actively explored functionalities include spins [4] , [5] , orbital states [6] or polarization [7] , [8] , [9] . In parallel, significant effort is focused on materials with ionically controlled electronic functionalities, including memristive and electroresistive devices [10] , [11] , [12] . Although yet unlikely to be a direct competition to mainstream semiconductor electronics, these alternatives offer advantages such as non-volatility and lower power consumption, coupling with optical and magnetic functionalities, access to continuum spectrum of computational variables, or quantum degrees of freedom. However, development of viable computational schemes requires implementation of devices to control the flow and ideally amplify the relevant computational variable. In semiconductor technology, this is exemplified by the development of transistor by Bell Labs team, an achievement made possible by harnessing the field effect in semiconductors [13] . Correspondingly, advancement of alternative computational schemes requires exploration of field effects between coupled functionalities. Here we demonstrate the ionic field effect during ferroelectric domain switching, leading to both standard and anomalous switching. Controlling field history leads to formation of complex domain morphologies, associated with violation of microscopic return point memory [14] , [15] . These studies potentially enable new generation of computational and data storage devices. Anomalous polarization switching in ferroelectrics We studied polarization reversal under the action of the electric field produced by conductive tip of scanning probe microscope (SPM) [16] , [17] . Similar SPM tip-induced polarization reversal process has been explored in different materials by multiple groups worldwide [17] , [18] , [19] , [20] , [21] , [22] , [23] . These studies provide detailed information on mechanisms and kinetics of polarization reversal process induced by the SPM tip, including shape and sizes of the formed domains [17] , [18] , [20] , [21] , [24] , kinetics of the switching and relaxation [25] , [26] , [27] , and the role of the external conditions on these processes [22] , [28] . In most cases, tip-induced local polarization reversal led to the formation of isolated domains. In the lithium niobate, domains usually had regular hexagonal or circular shape [17] , [22] , [29] . In some cases, shape of the domains contained partially backswitched areas in the centre and along the path of grounded tip [25] , [30] , [31] , [32] . Investigations were performed in the 20-μm-thick plate of single-crystalline congruent LiNbO 3 . Measurements have been done on Veeco Dimension SPM in the environmental cell in nitrogen atmosphere allowing for humidity control in the range from 0 to 90%. However, we should note here that humidity sensor used in our setup has high error level at low values of humidity (below 1%). Here and below humidity <1% will be labelled as 0%. Unipolar rectangular and bipolar triangular pulses with amplitude U sw =20–100 V and duration t sw =50–250 ms were applied to the tip. Resulted domain structures were visualized in single frequency and band excitation piezoresponse force microscopy (PFM) modes [33] , [34] , [35] . All SPM images of the domains in this study are presented in the combined piezoresponse signal: PR=R × sin(θ) , where R and θ are the amplitude and phase of piezoresponse, respectively. All measurements have been carried out on Z − polar surface. Imaging after switching on Z + surface did not reveal resulted domain. This fact can be attributed to compete backswitching due to ineffective screening. Unexpectedly, tip-induced polarization reversal by bipolar triangular pulses at 75% of relative humidity led to formation of the complex spatial inhomogeneous domain structures ( Fig. 1 ). Similar structures have been observed in lithium niobate after switching in homogeneous field at elevated temperatures [36] . Symmetry and size of the formed structures were strongly dependent on number of the switching cycles. For example, switching by the single triangular pulse led to formation of the small circular domain with radius ~50 nm ( Fig. 1a ). Increasing of the number of cycles led to formation of symmetric domain structure with typical size ~150 nm. Structures symmetry and size changed with increasing of the number of cycles. Formation of three secondary domains along crystallographic y axes ( Fig. 1b ) has been observed after two cycles. Further increasing of the cycles number led to formation of additional secondary domains ( Fig. 1c ) and their merging ( Fig. 1d ). Note that PFM amplitude is the same inside and outside of domains, indicative of classical ferroelectric behaviour. 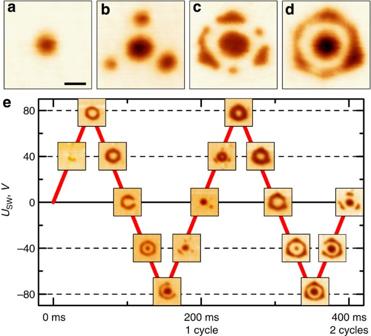Figure 1: Shapes of the domains formed after switching by sequence of bipolar triangular pulses. (a) 1, (b) 2, (c) 3 and (d) 5 complete cycles. (e) Domain shape evolution at different stages of the switching pulse. Relative humidityH=75% and pulse amplitudeUsw=80 V. Scale bar, 100 nm. Figure 1: Shapes of the domains formed after switching by sequence of bipolar triangular pulses. ( a ) 1, ( b ) 2, ( c ) 3 and ( d ) 5 complete cycles. ( e ) Domain shape evolution at different stages of the switching pulse. Relative humidity H =75% and pulse amplitude U sw =80 V. Scale bar, 100 nm. Full size image To explore the mechanism leading to formation of these complex patterns, the evolution of domain shape at different stages of applied triangular switching pulse was explored. Here the triangular wave was stopped at indicated point, the tip potential was reduced to zero when maintaining contact with the sample surface and the resultant domain structure was imaged by PFM. Visualization of the intermediate domain images allowed to reconstruct evolution of the domain shape during application of two bipolar triangular pulses is illustrated in Fig. 1e . These measurements demonstrated very unusual behaviour. Application of the electric field with the same direction as spontaneous polarization ( U sw >0 V) led to formation of the ring-shaped domains. In addition, application of the electric field with opposite direction led to normal switching with formation of circular domains. The subsequent cycling lead to the loss of stability of the ring domains, with the formation of well-defined satellites. To get further insight in the anomalous switching behaviour, polarization reversal induced by single pulses was explored. Rectangular pulses with amplitude U sw =±80 V and duration t sw =200 ms were used. Continuous acquisition of the piezoresponse signals during switching allowed determining the moment of polarization reversal ( Fig. 2 ). 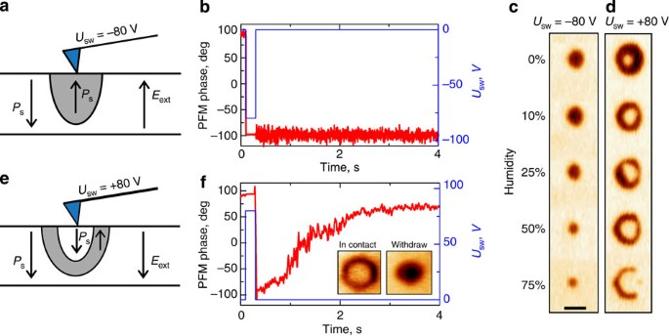Figure 2: Switching by single rectangular pulses. (a–c) Normal switching by field with opposite direction toPs; (d–f) field effect switching against to applied electric field. (a,e) Scheme of switching; (b,f) time dependencies of the PFM phase signal; (c,d) PFM image of the formed domains at different values of the relative humidity. Scale bar, 200 nm. Figure 2: Switching by single rectangular pulses. ( a – c ) Normal switching by field with opposite direction to P s ; ( d – f ) field effect switching against to applied electric field. ( a , e ) Scheme of switching; ( b , f ) time dependencies of the PFM phase signal; ( c , d ) PFM image of the formed domains at different values of the relative humidity. Scale bar, 200 nm. Full size image ‘Normal’ polarization reversal was observed after application of the electric field with direction opposite to P s ( Fig. 2a ). Phase of the piezoresponse changed on 180° instantly after application of the switching voltage and did not change after switching it off ( Fig. 2b ). Increasing of the amplitude signal during application of the bias is due to electrostatic interaction between sample surface and the tip. Further PFM visualization showed formation of the circular domains with radius ~50 nm ( Fig. 2c ). Unexpectedly, application of the nominally non-switching rectangular pulses with amplitude U sw =+80 V also lead to polarization reversal, as shown in Fig. 2e . This ‘abnormal’ polarization reversal occurs against applied electric field. However, in this case, phase flip (that is, switching event) is observed at the falling edge of the switching pulse ( Fig. 2f ) rather than during application of the field as is the case for normal switching. PFM visualization after abnormal switching showed formation of the ring-shaped domains with radius above 120 nm, significantly exceeding the size of the domains formed as a result of normal switching ( Fig. 2d ). To rationalize these observations, we speculate that the abnormal switching is induced by the redistribution of the screening charges on the surface and top layer of ferroelectric. On application of tip bias, applied electric filed along P s is screened by surface and bulk charges of the opposite sign. After switching the bias off, these accumulated sluggish charges produce electric field that induces polarization reversal nominally against the field. The ring shape of the domain can then be explained by back switching of polarization, as is directly confirmed by observed time dependencies of the piezoresponse signals ( Fig. 2f ). Phase flips instantly after termination of the pulse; however, in few seconds it relaxes to the initial value. Typical time of the phase relaxation was varied from milliseconds (in this case, phase did not flip at all) to dozen seconds. In all these cases, PFM imaging has shown formation of ring-shaped domains with approximately same sizes. This explanation was confirmed by the experiments when tip was withdrawn from the sample surface before termination of the switching pulse. In this case, formation of the solid domains oriented against the electric fields was observed ( Fig. 2f ), consistent with switching induced by the accumulated screening field. Similar behaviour has been observed by the number of scientific groups and has been attributed to charge injection [30] , [32] , [37] and ferroelastoelectric switching due to mechanical stress under the tip [31] . In this particular case, ferroelastic explanation is unlikely because the switching kinetics in our investigations was not dependent on the mechanical characteristics of the used tip and load on the tip, which is defined by the value of SPM set point parameter. At the same time, other papers described that phenomenon but have not explained it [38] . To separate surface and bulk screening, measurements have been performed as a function of humidity. For normal switching, the domain size decreases for larger humidity ( Fig. 2c ), the behaviour that can be explained by delocalization of the electric field due to the water meniscus in vicinity of the tip [39] . Abnormal switching led to formation of the rings with the same external size, while the area of the backswitched central zone decreased with humidity ( Fig. 2d ). These results mean that abnormal switching is not controlled by the surface state, although backswitching under the grounded tip is strongly affected by screening along the surface. These observations suggest that formation of the complex domain structures as shown in Fig. 1 can be generally represented as a superposition of several processes: 1 formation of the ring-shaped domain in the first half period ( U sw >0 V) of the switching pulse; 2 formation of the circular-shaped domain in the centre of the ring in the second half period ( U sw <0 V); 3 growth of the central domain and decay of the ring due to their interaction; 4 radial symmetry breaking of the ring-type domains giving rise to width modulation of the ring and formation of the satellites. Measurements showed that geometry, size and even symmetry of the domains produced by sequence of bipolar triangular pulses can be changed by varying of the set of control parameters: humidity, pulse amplitude and number of cycles ( Fig. 3 ). Switching at dry atmosphere ( H =0%) always led to the formation of solid circular-shaped domains, with size increasing with increasing of the cycle number ( Fig. 3a ). 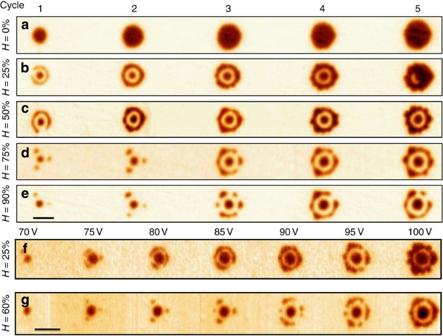Figure 3: Shapes of the domains formed at different values of humidity and amplitude. (a–e) Dependence of humidity and number of the cycles,Usw=80 V. (f,g) Dependence of pulse amplitude, two cycles in sequence. Scale bar, 250 nm (a,e), on– 500 nm (f,g). Figure 3: Shapes of the domains formed at different values of humidity and amplitude. ( a – e ) Dependence of humidity and number of the cycles, U sw =80 V. ( f , g ) Dependence of pulse amplitude, two cycles in sequence. Scale bar, 250 nm ( a , e ), on– 500 nm ( f , g ). Full size image Increasing of the humidity value up to 50% led to formation of the embedded structures (central domain and ring around it) ( Fig. 3b,c ). Symmetry of the external ring changed from regular hexagonal for one to three cycles to irregular forfour to five cycles. Similar symmetry breaking has been observed for high amplitudes of the switching pulse ( Fig. 3f,g ). Finally, increasing of the humidity above 50% leads to decay of the external ring and formation of the symmetric structures consisted of few secondary domains along crystallographic axes ( Fig. 3d,e,g ). Number of the domains and density of the structure decrease with increasing of the humidity. This surprisingly complex set of dynamic behaviours during multiple application of switching pulses as well as observation of anomalous switching against the applied field require consistent theoretical description. Below, we discuss some of the possible origins of anomalous switching and trace them to the ionic field effect on polarization switching. We further develop this analysis to explain the formation of the ring structures (radial instability) and subsequently the angular instability of the ring. Ionic field effect in ferroelectric switching To analyse the possible mechanisms of the normal and abnormal polarization switching, we note that the application of the bias to the tip leads both to the normal and radial electric field. Both components can be readily estimated in the effective charge approximation [40] , as plotted in Fig. 4 (see Supplementary Note 1 for details). The normal component of the tip field is maximal directly below the tip at ρ =0 and naturally leads to the formation of the central cylindrical domain under the tip in normal switching process (see schematics and coordinate system in Fig. 4a ). The radial component (1b) is zero at ρ =0 and has a sharp maximum at , where a * is effective tip radius. At distances ρ ⩾ a *, the radial field is higher than the normal one and scales as ρ −2 , while the normal component scales as ρ −3 . The resulting electric field at the surface becomes almost radial at large, ρ >2 a *, distances from the probe axis (see Fig. 4b ). The magnitudes of the characteristic fields can be estimated for the applied voltage of U =60 V, effective tip size a =50 nm, dielectric tip-surface gap of H =10 nm and dielectric anisotropy γ ≈0.8 as E tip (0,0)≈10 9 V m −1 . These extremely high fields common to voltage-modulated SPM experiments can readily induce ionic transport and electrochemical processes. 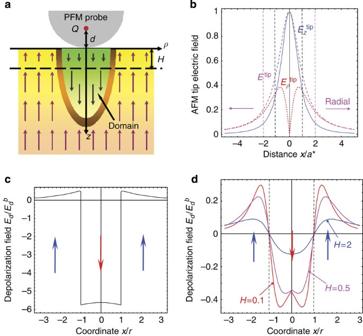Figure 4: Electric fields distribution. (a) Schematics and coordinate system. (b) SPM tip electric field components,and absolute valueEtip(ρ,0) normalized on the fieldU/a*. Applied voltageU=60 V, effective tip sizea*=50 nm,H=10 nm andγ≈0.8, we getEtip(0,0)≈109V m−1. Depolarization field created by a cylindrical domain of radiusrin the system ‘ferroelectric /tip/dry air’ (c) and ‘ferroelectric/tip/water meniscus’ at different ratioH/a(d). Figure 4: Electric fields distribution. ( a ) Schematics and coordinate system. ( b ) SPM tip electric field components , and absolute value E tip ( ρ ,0) normalized on the field U / a *. Applied voltage U =60 V, effective tip size a *=50 nm, H =10 nm and γ ≈0.8, we get E tip (0,0)≈10 9 V m −1 . Depolarization field created by a cylindrical domain of radius r in the system ‘ferroelectric /tip/dry air’ ( c ) and ‘ferroelectric/tip/water meniscus’ at different ratio H/a ( d ). Full size image The normal switching takes place when the tip charge is negative and the spontaneous polarization direction is downward from the ferroelectric surface. Note that although the process is nominally trivial (polarization orients along the electric field), it implicitly implies ready availability and high mobility of screening charges. For the case of the negative polarization bound charge, the screening is initially realized by highly mobile protons, H + . In this case, rapid polarization reversal takes place just below the tip (that is, inside the circle ρ < a *) and immediately after the switching the protons are moved away from the region ρ < a *. The reversed polarization charge is almost simultaneously screened by the free electrons injected from the tip. In the presence of water layer, the screening by electrons is eventually substituted by slower, but more effective screening by OH − . Note that relatively slower mobility of hydroxyls leads to partial backswitching once the tip bias is turned off, but still is in contact with the surface, as proposed by ref. 41 . The abnormal switching takes place when the tip charge is positive and the spontaneous polarization direction is downward from the ferroelectric surface. The screening of ferroelectric polarization end (negative bound charge) below the tip is realized by the protons (as in the previous ‘normal’ case), but in the case positively charged protons can rapidly move far away from the tip and the surface ρ <3 a* becomes unscreened, because there are no excess of the free electrons from the tip. The application of positive tip bias further induces accumulation of sluggish negatively charged OH − below the tip. Note that OH − groups cannot penetrate into the LiNbO 3 and are non-volatile; thus, formally they are mobile mainly in transverse directions. This accumulation of negative charges occurs while the tip is biased, U >0. When the voltage is off ( U =0), the remaining slow negative charges induce the polarization switching. The size of the switched domain is controlled by the initial lateral field distribution, that is, the effective tip size. Radial instability and formation of the ring structures Formation of the ring domain structures has been observed as a result of abnormal polarization reversal. Experiments showed that ring-like shape is due to backswitching phenomenon in the area under the tip. Typical time of the backswitching varied from microseconds to tens of seconds. The additional factor that can stabilize the ring structures is the depolarization field effect as introduced in ref. 23 . Here, the depolarization field created by a cylindrical domain in the system ‘ferroelectric surface/tip/water meniscus’ is much smaller than in the dry conditions and has maxima at definite distance from the domain wall (DW; details of the field calculations are listed in refs 23 , 42 ), that is, in a ring around existing domain to the appearance of the screening charge ring (see Fig. 4c,d ). We note however that this can stabilize the ring structure, but cannot explain their formation. Angular instability of the ring Most remarkable are the observations of the angular instabilities of the ring that can lead to formation of threefold satellites oriented along y crystallographic axis, sixfold satellites, and striations, and even lower symmetry features. This broad spectrum of behaviours suggests the presence of several competing instabilities. Here we consider thermodynamic effects related to the angular instability formation during growth, thermodynamic instability of the ring during relaxation, instabilities related to transport of screening charges and dynamic instabilities of meniscus. To analyse the thermodynamics of domain formation, we note that non-ferroelectric transverse components of polarization can be regarded proportional to the electric field: , while the ferroelectric z component is in the first approximation, where E d is the depolarization electric field (see Supplementary Note 2 for details). Electrostriction couples the polarization components to the strain, u ij = Q ijkl P k P l , where Q ijkl is the electrostriction stress tensor. For LiNbO 3 with 3 m symmetry, the strain leads to the renormalization of coefficient α 3 in the Landau-Ginzburg-Devonshire theory free energy term, , namely α 3 = α 0 +2 q 31 ( u 11 + u 22 )+2 q 33 u 33 , where q ijkl is the electrostriction strain tensor. The evident form of the α 3 ( ρ , z ) variation caused by the ‘bare’ tip field is X-profile of the radial variation is shown in Fig. 5a at y =0, z =0 and LiNbO 3 parameters at room temperature. The variation δα r is indeed small in comparison with α 3 ( ρ , z ) and thus can act only as a source of the polarization instability in the ring, as will be demonstrated below. 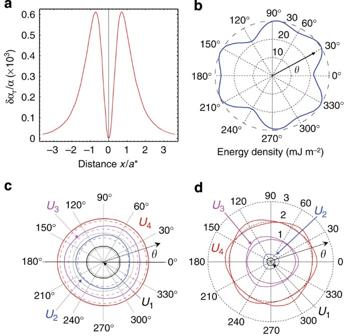Figure 5: Theoretical calculations of the domain shape. (a) X-profile of the radial variationcalculated atz=y=0, and room temperature LNO parametersε11=84,ε33=39,Q31=−0.003 m4/C2,Q33=+0.016 m4/C2,q31=−0.216 N × 109N × m2/C2,q33=+1.848 × 109N × m2/C2,,α0=2.012 × 109N × m2/C2,43U=50 V, effective tip sizea*=25 nm. (b) Angular dependence (polar plot) of the 180° DW energy density. Domain shape at different voltagesU1<U2<U3<U4in the system ‘ferroelectric/tip/dry air’ (c) and ‘ferroelectric /tip/water meniscus’ (d). Figure 5: Theoretical calculations of the domain shape. ( a ) X-profile of the radial variation calculated at z=y= 0, and room temperature LNO parameters ε 11 =84, ε 33 =39, Q 31 =−0.003 m 4 /C 2 , Q 33 =+0.016 m 4 /C 2 , q 31 =−0.216 N × 10 9 N × m 2 /C 2 , q 33 =+1.848 × 10 9 N × m 2 /C 2 , , α 0 =2.012 × 10 9 N × m 2 /C 2 , [43] U =50 V, effective tip size a *=25 nm. ( b ) Angular dependence (polar plot) of the 180° DW energy density. Domain shape at different voltages U 1 < U 2 < U 3 < U 4 in the system ‘ferroelectric/tip/dry air’ ( c ) and ‘ferroelectric /tip/water meniscus’ ( d ). Full size image Relaxation of the ring due to interaction with growing central domain can be explained by the mechanism described in previous section for domain growth. It is very important for further consideration fact Scrymgeour et al . [43] have shown the 180-degree DW energy in LiNbO 3 is essentially anisotropic with respect to the mutual orientation of the wall and crystallographic axes. The anisotropy is defined by the intrinsic anisotropy of the electrostriction coefficients that in the local coordinate system linked to the DW can be interpolated as where θ is the polar angle in the local coordinate system and χ i are the anisotropy coefficients corresponding to the trigonal or hexagonal symmetry. Angular dependence of the 180° DW energy density is shown in Fig. 5b . The ferroelectric polarization P 3 obeys to the time-dependent Landau-Ginzburg-Devonshire equation: where α 3 = α (1+ χ 1 sin 2 (3 θ /2)+ χ 2 sin 2 (3 θ )) and |χ i | ≪ 1 in accordance with equations (2) and (3). To look for the condition of the ring-type instability, equation (4) was linearized in the vicinity of near-surface value P eff as P 3 = P eff + δP 3 with zero boundary conditions δP 3 ( r )=0, δP 3 ( R )=0, 0< r < R . As it was mentioned in the subsection 1, in the wet ambient (humidity H >30–40%) the value of P eff can be essentially smaller than the LiNbO 3 spontaneous polarization P S in the effective layer enriched by protons. In dry ambient H =0 and P eff =± P S . The condition of the absolute ring-type instability (see Supplementary Notes 3 and 4 for details): As α is negative in the ferroelectric phase, g is positive and wave number are real. The ring-type instability given by equation (5) can exist in the region 0< r < R only if . This shows us that the presence of wet ambient creating the effective layer of thickness H with suppressed polarization is critically important for the ring-type instability appearance. Note that equation (5) indicates the possibility of the ring-type domain instability but as any linearized solution cannot be used for quantitative modelling of domain shape. Equilibrium domain shapes in the system ‘ferroelectric/tip/dry air’ and ‘ferroelectric /tip/water meniscus’ were modelled using the nonlinear master equation with the surface tension term included and allowing for equation (4) (see Supplementary Note 5 for details). Results at different voltages U 1 < U 2 < U 3 < U 4 are shown in Fig. 5c,d correspondingly. In the case of ‘dry’ ambient the shape is almost circular, in the ‘wet’ ambient the trigonal or hexagonal angular instability appears. The formation of the low-symmetry irregular features may be indicative of the classical Mullins–Sekerka or viscous fingering-type instabilities [44] , [45] controlled by the transport of the screening species to the growing domains. Here we note that the maximum instabilities are observed for high values of relative humidity, at which the surface ionic transport can be expected to be most facile. Hence, this mechanism is unlikely to account for observed behaviour. In addition, irregular shape of the domains can be attributed to the lack of the stability of the water meniscus at high values of the electric field. Application of the electric field to conductive SPM tip leads to polarization of the water and injection of the charges into the meniscus. Both phenomena cause repulsive force, which aims at the meniscus stretching. On the other hand, this repulsive force is compensated by compressive surface tension force. Ratio of these two forces defines stability of the water meniscus. Exceeding of the threshold bias value leads to lack of the meniscus shape stability and can explain irregularity of the domain shapes at high biases. Rough estimations can be used to find critical value of the voltage applied to free water droplet. Electric potential of the droplet is produced by charges distributed by the external droplet surface. In this case, electrostatic forces act on stretching of the droplet. In the approximation of spherical droplet with radius R d and applied potential U , the pressure produced by electrostatic forces is equal: . On the other hand, surface tension forces squeeze the droplet and produce the pressure p st =2/ γR d , where γ is the constant of surface tension. In this case, critical value of the voltage U cr is defined by expression p es =p st : . Estimations for droplet with radius R d =100 nm gives critical value of the applied voltage ~50 V. Of course this rough estimation can be used only to get order of magnitude of the real critical voltage applied to the real water meniscus. Moreover, this value is close to the biases used in the experiments. Data encoding in domain shape We further explore feasibility of data encoding in the domain shape. Experimentally data coding can be realized as a switching by sequence of positive and negative triangular pulses (positive codes ‘1’, negative − ‘0’), leading to formation of isolated domains. Example of experimentally realized 3-bit coding is presented in Fig. 6 . Switching has been carried out by combination of three positive and negative pulses. Switching was repeated three times in each point (nine pulses have been applied in total). As one can see from eight possible combinations, at least seven can be visually distinguished by shape and size of the resulted domain. Hence, the shape and size of the domain keep information about used sequence. Furthermore, explored phenomena can be used as a simplest computational device. Size and shape of the domain depend on the number of applied pulses, so resulted domain image can be used for extracting information of few independent sequences applied in the same point. For example, this approach can be used for sum operation as offered inref. [46] on the basis of phase change materials. 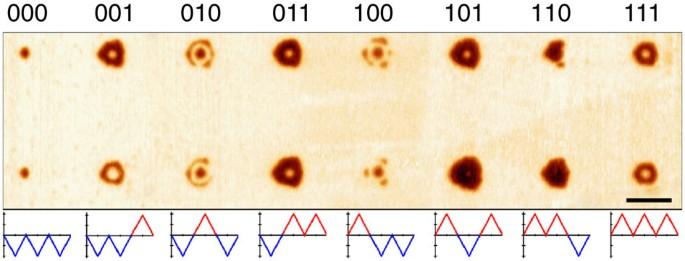Figure 6: Domain shape data coding. Domains formed as a result of switching by different sequences of positive and negative triangular pulses.Usw=80 V, three cycles. Scale bar, 500 nm. Figure 6: Domain shape data coding. Domains formed as a result of switching by different sequences of positive and negative triangular pulses. U sw =80 V, three cycles. Scale bar, 500 nm. Full size image To summarize, we explored formation of the complex symmetric domain structures consisting of separate domains as a result of the local polarization reversal by sequences of bipolar triangular pulses. Investigation of the domain shape evolution and model experiments by single rectangular pulses allowed describe process of them formation as a multistage process. One part of which is ‘abnormal’ polarization reversal against applied electric field has been studied and explained by switching under the action of the surface and bulk charges in the sample. Measurements at different values of relative humidity showed that kinetics of polarization reversal by bipolar triangular pulses, shape and even symmetry of the formed structures can be controlled by the set of parameters: humidity, amplitude and number of cycles. Furthermore, the interplay between switching and ionic dynamics allows information storage and logical operation on a single domain level. Finally, we note that universality of screening phenomena for ferroelectrics suggest that similar phenomena can occur in other materials, as indeed supported by observation of non-cylindrical domains is other ferroelectric and even relaxor-ferroelectric materials [31] , [32] , [38] . How to cite this article: Ievlev, A. V. et al . Ionic field effect and memristive phenomena in single-point ferroelectric domain switching. Nat. Commun. 5:4545 doi: 10.1038/ncomms5545 (2014).